Accumulation of differentiating intestinal stem cell progenies drives tumorigenesis Stem cell self-renewal and differentiation are coordinated to maintain tissue homeostasis and prevent cancer. Mutations causing stem cell proliferation are traditionally the focus of cancer studies. However, the contribution of the differentiating stem cell progenies in tumorigenesis is poorly characterized. Here we report that loss of the SOX transcription factor, Sox21a, blocks the differentiation programme of enteroblast (EB), the intestinal stem cell progeny in the adult Drosophila midgut. This results in EB accumulation and formation of tumours . Sox21a tumour initiation and growth involve stem cell proliferation induced by the unpaired 2 mitogen released from accumulating EBs generating a feed-forward loop. EBs found in the tumours are heterogeneous and grow towards the intestinal lumen. Sox21a tumours modulate their environment by secreting matrix metalloproteinase and reactive oxygen species. Enterocytes surrounding the tumours are eliminated through delamination allowing tumour progression, a process requiring JNK activation. Our data highlight the tumorigenic properties of transit differentiating cells. Maintenance of tissue homeostasis in the adulthood requires precise coordination of stem cell renewal and differentiation. Deregulation of these processes can lead to cancer. Stem cells live in a microenvironment and continuously receive signals from neighbouring heterologous cells composing the niche [1] . Stem cell niches are complex, heterotypic and dynamic structures [2] . Over the past few years, considerable progress has been made in elucidating how different niche factor promotes stem cell maintenance during homeostasis and contributes to tissue regeneration upon damage [3] , [4] . Stem cells usually divide asymmetrically to generate a self-renewing stem cell and a differentiating progenitor (or transit amplifying cell), which will eventually generate differentiated cells [5] . Recent studies in flies and mammals have begun to establish that these differentiating progenitors are not simply a passive intermediate between stem cell and differentiated cells, but play active roles in regulating stem cell activity and regeneration [6] , [7] , [8] , [9] , [10] . Loss of proper differentiation is an important feature and likely a driver of cancer development [11] . Historically, mechanistic studies of human cancers and regenerative medicine have focused almost exclusively on stem cells [2] , [12] . The roles of the differentiating stem cell progeny in tumorigenesis remain largely unexplored [3] , [10] . In this study, we analyse how a defect in the differentiating program of stem cell progenies leads to tumours in the adult Drosophila intestine. The adult intestine is continuously replenished by multipotent intestinal stem cells (ISCs) both in flies and mammals [4] , [12] , [13] . In the Drosophila midgut, ISCs differentiate into either large absorptive enterocytes or secretory enteroendocrine cells. This process involves an intermediate differentiating cell called the enteroblast (EB; Fig. 1a ) [14] , [15] , [16] , analogous to the transit amplifying cell in mammalian intestines [17] . In this study, we show that Sox21a , a gene encoding a transcription factor of the SOX family, is required for EBs to become fully differentiated cells. Flies lacking Sox21a are viable but progressively develop intestinal tumours composed mainly of EBs. Using Drosophila genetics, we have provided a comprehensive dissection of cell–cell interactions that underlie the EB tumour initiation and progression as a result of this differentiation defect. Our data highlight a driving role of differentiating stem cell progenies in tumorigenesis. While the implication of stem cells in cancer has been the focus of intensive research, our data pinpoint the tumorigenic properties of transit differentiating cells. We speculate that the plasticity of these differentiating progenitors underlies their cancerous properties. 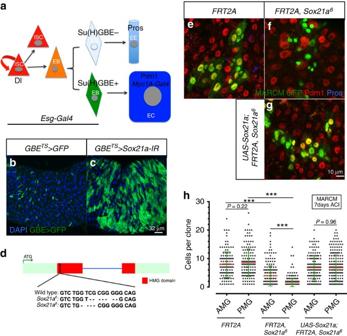Figure 1:Sox21ais required for EB differentiation. (a) Model of intestinal stem cell (ISC) lineages. The markers used in this study areDelta(Dl)-GFP/lacZ: ISC,escargot(esg)-Gal4or Armadillo (Arm): progenitors (ISC+EB),Su(H)GBE-Gal4/lacZ: EB, Prospero (Pros): enteroendocrine cells (EE), Pdm1 orMyo1A-Gal4: enterocytes (EC). (b,c) Anterior midgut (AMG) of control fly and fly expressing aSox21a-RNAitransgene in EBs for 14 days at 29 °C. Nuclei are stained for 4′,6-diamidino-2-phenylindole (DAPI; blue). EBs expressGBE>GFP(green). (d) Schematic representation ofSox21amutant alleles generated with CRISPR/Cas9 method. Sequences deleted are represented with dashed line. (e-g) Representative images of GFP-labelled MARCM clones from AMG of flies with indicated genotypes at 7 days after clone induction (ACI). Pdm1 (red) and Pros (blue). (h), Quantification of MARCM clone size for both AMG and posterior midgut (PMG) of experiments ine-g. Mean and s.e.m. are shown inh, with 136, 160, 221, 324, 166 and 274 clones (left to right) scored from 16 flies as a representative of three independent experiments.Pvalues from Student’st-test (*P<0.05; **P<0.01; ***P<0.001). One representative image from 16 midguts tested in one experiment, which was repeated three times, is shown inb,cande-g. Figure 1: Sox21a is required for EB differentiation. ( a ) Model of intestinal stem cell (ISC) lineages. The markers used in this study are Delta ( Dl ) -GFP/lacZ : ISC, escargot ( esg )- Gal4 or Armadillo (Arm): progenitors (ISC+EB), Su(H)GBE-Gal4/lacZ : EB, Prospero (Pros): enteroendocrine cells (EE), Pdm1 or Myo1A-Gal4 : enterocytes (EC). ( b , c ) Anterior midgut (AMG) of control fly and fly expressing a Sox21a-RNAi transgene in EBs for 14 days at 29 °C. Nuclei are stained for 4′,6-diamidino-2-phenylindole (DAPI; blue). EBs express GBE>GFP (green). ( d ) Schematic representation of Sox21a mutant alleles generated with CRISPR/Cas9 method. Sequences deleted are represented with dashed line. ( e-g ) Representative images of GFP-labelled MARCM clones from AMG of flies with indicated genotypes at 7 days after clone induction (ACI). Pdm1 (red) and Pros (blue). ( h ), Quantification of MARCM clone size for both AMG and posterior midgut (PMG) of experiments in e - g . Mean and s.e.m. are shown in h , with 136, 160, 221, 324, 166 and 274 clones (left to right) scored from 16 flies as a representative of three independent experiments. P values from Student’s t -test (* P <0.05; ** P <0.01; *** P <0.001). One representative image from 16 midguts tested in one experiment, which was repeated three times, is shown in b , c and e-g . Full size image Sox21a is necessary for EB differentiation In an RNA interference (RNAi) screen for factors regulating stem cell differentiation, we identified Sox21a , a gene encoding a transcription factor of the SOX family with homologues implicated in stem cell regulation in mammals [18] . Silencing Sox21a with two independent RNAi constructs specifically in EBs using the conditional, temperature-sensitive Su(H)GBE-Gal4 UAS-GFP tub-Gal80 TS system (hereafter referred to as GBE TS ) [19] led to the accumulation of EBs in the adult ( Fig. 1b,c ; Supplementary Fig. 1a–c ). Consistent with this, Sox21a is specifically enriched in the midgut of adult Drosophila ( Supplementary Fig. 1d ). Moreover, examination of the cis -regulatory sequences of the Sox21a gene also revealed an intronic enhancer that drives reporter expression in both ISCs and EBs (referred to as progenitors; Supplementary Fig. 1e–h ). The expression pattern driven by this enhancer is homogenous from the anterior to the posterior midgut, and is identical to the expression of Escargot (Esg), a transcription factor with well-defined expression in progenitors [20] . To further study the function of Sox21a, we have generated two Sox21a mutations using CRISPR/Cas9-mediated genome editing [21] . Both mutants carry a small deletion in the DNA-binding domain of Sox21a, the HMG domain, resulting in reading frameshift and premature stop ( Fig. 1d ). Thus, these alleles should be considered as null alleles. Strikingly, Sox21a mutant flies are viable and fertile with no apparent defects. To confirm the role of Sox21a in EB differentiation, we performed lineage tracing using mosaic analysis with a repressible cell marker technique (MARCM) [22] . While the wild-type clones (positively marked by green fluorescent protein (GFP)) contain both enterocytes and enteroendocrine cells, cells in Sox21a mutant clones along the whole midgut remained undifferentiated, as revealed by the absence of GFP-positive cells expressing the enterocyte marker Pdm1 or the enteroendocrine cell marker Prospero ( Fig. 1e,f ). This differentiation defect is rescued by overexpressing Sox21a in the mutant clones ( Fig. 1g ). Quantification of clone size indicated that the Sox21a mutation reduces ISC division with a stronger effect in the posterior compared with the anterior midgut ( Fig. 1h ). Sox21a mutant clones generated in the posterior midgut barely grew, indicating a mandatory function of Sox21a for ISC division in the posterior midgut. In contrast, the existence of large Sox21a mutant clones in the anterior midgut indicates that Sox21a promotes to some extent stem cell division in this region but is less essential. The presence of a wild-type copy of Sox21a in the mutant clones also restored normal ISC division ( Fig. 1h ). To further confirm the differential impact of Sox21a on ISC division in the anterior and posterior regions, we compared ISC proliferation rate in wild-type and Sox21a mutant flies overexpressing the JAK/STAT ligand unpaired 2 (Upd2) in the enterocytes with Myo1A-Gal4 UAS-GFP tub-Gal80 TS system (hereafter referred to as Myo1A TS ) [23] . Unpaired are secreted proteins that have been shown to be potent inducers of ISC proliferation by activating JAK/SAT signalling in ISCs [23] , [24] . Overexpressing Upd2 strongly increased the number of mitotic ISCs in both the anterior and the posterior midgut in wild-type flies as revealed by the phospho-Histone H3 (PH3, a mitotic marker) count. In contrast, overexpressing Upd2 only increased the mitotic index in the anterior midgut of Sox21a mutant ( Supplementary Fig. 4o,p ). Collectively, our data show that Sox21a is essential for the differentiation of EBs into mature intestinal cells along the entire midgut. Its effect on ISC proliferation is more pronounced in the posterior midgut compared with the anterior midgut. Overexpression of Sox21a drives EB differentiation Since Sox21a is required to generate differentiated cells, we hypothesized that overexpressing this factor might force the progenitor cells to differentiate into mature intestinal cells. To test this, we created transgenic lines that enable its overexpression via the GAL4/UAS system ( Supplementary Fig. 1g ). Strikingly, overexpressing Sox21a in the progenitor cells with esg-Gal4 UAS-GFP tub-Gal80 TS system (hereafter referred to as esg TS ) [15] was sufficient to induce their differentiation into enterocytes and cause the loss of progenitors ( Fig. 2a–c ). Although Sox21a is required for the differentiation of both enterocytes and enteroendocrine cells, Sox21a overexpression induced progenitors to differentiate into enterocytes (Pdm1 positive and polyploid), but not enteroendocrine cells (Pros positive; Supplementary Fig. 2a,b ). To further delineate the role of Sox21a in progenitor differentiation, we overexpressed Sox21a either specifically in EBs using GBE TS or in ISCs using Dl-Gal4 UAS-GFP tub-Gal80 TS ( Dl TS ) [19] . EBs were normally detected as small-nucleated cells with a polarized cell shape ( Fig. 2d ). Overexpressing Sox21a in EBs for 4 days transformed most of them into large polyploid and round-shaped cells, indicative of a transformation into enterocyte ( Fig. 2e,f ). In contrast, overexpressing Sox21a with Dl TS in ISCs for 6 days did not induce ISC differentiation ( Supplementary Fig. 2c,d ). Using other insertions of the UAS-Sox21a transgene, we sometimes observed clusters of two to four ISCs (positive for Dl-lacZ ) when overexpressing Sox21a using esg TS ( Supplementary Fig. 2e,f ). Thus, besides inducing progenitor cells to differentiate, Sox21a may also have a role in stem cell division. We conclude that Sox21a is a critical factor required for the transition from EBs to mature intestinal cells in the adult midgut. 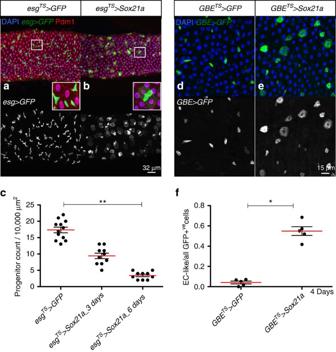Figure 2:Sox21ais sufficient to drive differentiation. (a,b) AMG of flies overexpressing GFP (control,a) orSox21a(b) in progenitor cells usingesgTSdriver for 2 days at 29 °C.esg>GFPchannel is also shown. Insets show a high-magnification view. Pdm1 staining is shown in red. (c) Quantification of the number of progenitor cells in a 10,000-μm2area in AMG of control and overexpressingSox21afor 3 and 6 days (n=12, 10 and 10, respectively). (d,e) AMG of flies overexpressing GFP (control,d) orSox21a(e) in EBs usingGBETSdriver for 4 days at 29 °C.GBE>GFPchannel is also shown. (f) Quantification of the ratio of newly formed EC-like cells to all the GFP-positive cells in AMG of control and overexpressingSox21afor 4 days (n=5). Error bars indicate s.e.m. (c,f).Pvalues from Student’st-test (*P<0.05; **P<0.01; ***P<0.001) are shown incandf, and the results represent three independent experiments. One representative image from 12 midguts tested in one experiment, which was repeated three times, is shown ina,b,dande. Figure 2: Sox21a is sufficient to drive differentiation. ( a , b ) AMG of flies overexpressing GFP (control, a ) or Sox21a ( b ) in progenitor cells using esg TS driver for 2 days at 29 °C. esg>GFP channel is also shown. Insets show a high-magnification view. Pdm1 staining is shown in red. ( c ) Quantification of the number of progenitor cells in a 10,000-μm 2 area in AMG of control and overexpressing Sox21a for 3 and 6 days ( n =12, 10 and 10, respectively). ( d , e ) AMG of flies overexpressing GFP (control, d ) or Sox21a ( e ) in EBs using GBE TS driver for 4 days at 29 °C. GBE>GFP channel is also shown. ( f ) Quantification of the ratio of newly formed EC-like cells to all the GFP-positive cells in AMG of control and overexpressing Sox21a for 4 days ( n =5). Error bars indicate s.e.m. ( c , f ). P values from Student’s t -test (* P <0.05; ** P <0.01; *** P <0.001) are shown in c and f , and the results represent three independent experiments. One representative image from 12 midguts tested in one experiment, which was repeated three times, is shown in a , b , d and e . Full size image Sox21a functions downstream of the JAK/STAT pathway The JAK/STAT pathway plays a major role in ISC proliferation and differentiation in Drosophila [23] , [25] . We therefore explored the relationship between Sox21a and JAK/STAT in stem cell differentiation. Quantitative reverse transcription–PCR (qRT–PCR) experiments showed that Sox21a expression is regulated by the JAK/STAT signalling pathway. Sox21a expression in the midgut was lower when Stat92E was silenced by RNAi using the esg TS driver and was higher when expressing a gain-of-function allele of JAK ( hop tumL ; Supplementary Fig. 2g ). Previous study has shown that MARCM clone cells mutant for Stat92E were also negative for enterocyte marker Pdm1 ( Supplementary Fig. 2h ), consistent with a mandatory role of JAK/STAT in progenitor differentiation [23] , [25] . Moreover, overexpression of Sox21a restored the expression of the enterocyte marker Pdm1 in Stat92E null mutant clones, confirming the role of Sox21a as a major downstream effector of this pathway in mediating differentiation ( Supplementary Fig. 2i ). The position of Sox21a downstream of the JAK/STAT pathway and its role in EB differentiation were reinforced by two other observations. First, the expression of esg and its regulator miR-8 , two genes encoding factors regulating the progenitor identity [16] , [20] , was not affected in Sox21a flies ( Fig. 3a,b ; Supplementary Fig. 3a,b ). Second, the expression of Pdm1, a transcription factor specifically expressed in enterocyte [20] , was downregulated in Sox21a mutant EBs (see RNA sequencing (RNA-seq) experiment, described below). 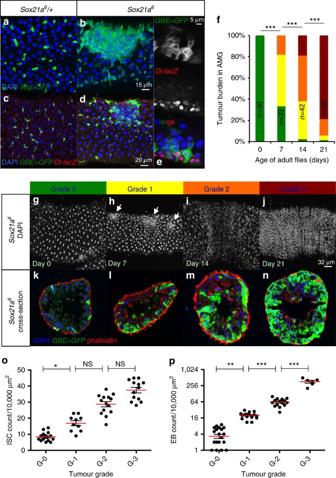Figure 3: Characterization ofSox21atumours. (a–d) AMG of 10-day-oldSox21a/+(control,a,c) andSox21aflies (b,d), carrying eitheresg>GFP(a,b) orDl-lacZandGBE>GFP(b,d). (e) A confocal section to show the basal–apical (bottom-up) organization of ISCs and EBs inSox21afly. (f) Quantification of tumour burden ofSox21aflies at the indicated age at 25 °C (n=30, 33, 42 and 50, respectively). (g–n) Superficial view (g–j, DAPI) and cross-sections (k–n, EBs in green, phalloidin in red) of intestines fromSox21aflies. Tumour grade is colour-coded from green (grade 0) to red (grade 3). Arrows indicate small clusters of progenitor cells (h). (o,p) Quantification of the number of ISCs (o) and EBs (p) in a 10, 000-μm2area from tumours of different grade (n=16, 10, 14 and 13, respectively ino;n=24, 17, 15 and 6, respectively inp). Error bars indicate s.e.m. (o,p).Pvalues inffromχ2-test, and inoandpfrom Student’st-test (*P<0.05; **P<0.01; ***P<0.001; NS, not significant). Each plot (f,o,p) is representative of three biological replicates. Each image shown ina–eandg–nrepresents 25 flies tested in one experiment and repeated three times. Figure 3: Characterization of Sox21a tumours. ( a – d ) AMG of 10-day-old Sox21a/+ (control, a , c ) and Sox21a flies ( b , d ), carrying either esg>GFP ( a , b ) or Dl-lacZ and GBE>GFP ( b , d ). ( e ) A confocal section to show the basal–apical (bottom-up) organization of ISCs and EBs in Sox21a fly. ( f ) Quantification of tumour burden of Sox21a flies at the indicated age at 25 °C ( n =30, 33, 42 and 50, respectively). ( g – n ) Superficial view ( g – j , DAPI) and cross-sections ( k – n , EBs in green, phalloidin in red) of intestines from Sox21a flies. Tumour grade is colour-coded from green (grade 0) to red (grade 3). Arrows indicate small clusters of progenitor cells ( h ). ( o , p ) Quantification of the number of ISCs ( o ) and EBs ( p ) in a 10, 000-μm 2 area from tumours of different grade ( n =16, 10, 14 and 13, respectively in o ; n =24, 17, 15 and 6, respectively in p ). Error bars indicate s.e.m. ( o , p ). P values in f from χ 2 -test, and in o and p from Student’s t -test (* P <0.05; ** P <0.01; *** P <0.001; NS, not significant). Each plot ( f , o , p ) is representative of three biological replicates. Each image shown in a – e and g – n represents 25 flies tested in one experiment and repeated three times. Full size image Accumulation of EBs and formation of tumour in Sox21a flies A striking feature of Sox21a flies is the presence of large clusters of progenitors in the anterior but not the posterior midgut ( Supplementary Fig. 4a–n ). This regional difference is not surprising, since the Sox21a mutation has a differential effect on the ISC division rate in the anterior and posterior midgut. We have focused our subsequent studies on the anterior midgut to analyse the formation of these clusters. They contain both ISCs and EBs, but progressively become dominated by EBs, consistent with the function of Sox21a in EB differentiation ( Fig. 3a–d ; Supplementary Fig. 5a–h ). Similar to wild-type midgut, ISCs are localized basally, while EBs are found more apically towards the lumen in Sox21a mutant cluster ( Fig. 3e ). These clusters increase in size over time and grow towards the intestinal lumen, behaving like tumours ( Fig. 3g–n ; Supplementary Fig. 5a–d ). To quantify the tumour burden in individual midgut, we classified the tumours into four grades ranging from 0 to 3 based on their size and overgrowth ( Fig. 3g–n ; Supplementary Fig. 5a–d ; see method part for additional information on the grading criteria). After 3 weeks at 25 °C, most Sox21a mutant flies contain at least one grade 3 tumour ( Fig. 3f ). Quantification of ISC and EB number in the tumour revealed a nearly linear increase of ISCs but an exponential increase of EBs ( Fig. 3o,p ; Supplementary Fig. 5a–d,e–h ). This suggests that ISCs in Sox21a tumours are still functional and most likely divide asymmetrically to generate another self-renewing ISC and an EB blocked at this stage [26] , [27] . Sox21a tumour growth relies on ISC division We next explored the mechanisms by which a simple defect in the differentiation program of EBs leads to tumour formation. ISCs are the only proliferating cells in the midgut in normal conditions [17] . Although a study has reported that a small portion of EBs (<5%) displays mitotic activity upon enteric Pseudomonas entomophila infection, EBs do not divide under basal conditions [17] . Using PH3 staining, we analysed the identity of mitotic cells in Sox21a mutant expressing a GBE>GFP to mark EBs. While we detected many ISCs undergoing mitosis, no mitotic EB was observed ( n >100; Supplementary Fig. 6a ). We next explored whether tumour growth in Sox21a flies is sustained by stem cell division. Drosophila ISC division relies on the epidermal growth factor receptor (EGFR) signalling [28] . Blocking this pathway by expressing a dominant-negative form of EGFR in progenitors of Sox21a flies suppressed the formation of tumour ( Supplementary Fig. 6b–d ). The ingestion of enteric bacteria was previously shown to stimulate ISC proliferation in Drosophila and promotes tumorigenesis in other models [29] . Similarly, stimulating ISC proliferation by infecting Sox21a flies with bacteria increased the size and the numbers of tumours ( Supplementary Fig. 6e–g ). These observations indicate that ISC proliferation is essential for Sox21a tumour formation. This dependence on stem cell division again explains why tumours are only found in the anterior midgut but not the posterior midgut where Sox21a is required for both EB differentiation and ISC division. Interestingly, ISC proliferation was markedly increased in the neighbourhood of Sox21a tumours ( Supplementary Fig. 7a ). Consistent with this, use of 10xStat-GFP D reporter gene reveals higher JAK/STAT activity in the tumour ( Fig. 4a ). In addition, Sox21a mutant cells generated via MARCM triggered Ras/MAPK signalling in neighbouring wild-type cells, as revealed by a staining of phosphorylated ERK (dpERK) ( Fig. 4b ). Thus, Sox21a mutant cells induce a local hyperplasia by stimulating division in adjacent ISCs ( Supplementary Fig. 7b ). This suggests that EBs composing Sox21a tumours send a signal to neighbouring ISCs to drive their proliferation. 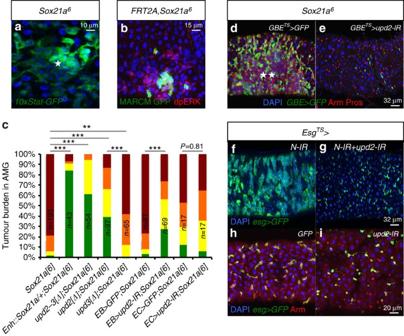Figure 4: EB-derivedupd2is essential for tumour growth and ISC maintenance. (a) AMG of 10-day-oldSox21aflies stained for10xSTAT-GFPD(green) shows increased JAK/STAT activity in the tumour (indicated by a star). (b) AMG containing GFP-labelledSox21amutant clone stained for dpERK (red) at 16 days ACI. dpERK staining is observed around theSox21aclone. (c) Tumour burden of flies with the indicated genotypes kept at 25 °C (mutant analysis) or 29 °C (overexpression analysis) for 21 days.Enh::Sox21ais a rescue construct withSox21aunder the control of its own enhancer sequence. ‘EB>’ refers to the EB driverGBETS, and ‘EC>’ refers to the enterocyte driverMyo1ATS. Numbers of flies scored for each genotype are indicated. (d,e) Expressing GFP (d, control) orupd2-RNAi(e) in EBs ofSox21aflies placed for 21 days at 29 °C. Gut was stained with Armadillo (Arm; red, plasma membrane for progenitors) and Prospero (Pros, red, nuclear, for enteroendocrine cells). EBs are marked byGBE>GFP(green). (f-g) AMG of flies depleted forNotch(N) alone (f) or in combination withupd2(g) for 4 days at 29 °C. The expression ofupd2-IRin progenitors reduced tumour formation. (h,i) AMG of flies expressing GFP (control,h) orupd2-RNAi(i) in the progenitor cells using theesgTSdriver for 14 days at 29 °C shows thatupd2is required for basal stem cell maintenance. Progenitors are shown byesg>GFPin green (f–i) and by Arm immunostaining (h,i).Pvalues inc(repeated three times) fromχ2-test (*P<0.05; **P<0.01; ***P<0.001). Each other individual image shown ina,band (d–i) represents 20 flies tested in one experiment repeated three times. Figure 4: EB-derived upd2 is essential for tumour growth and ISC maintenance. ( a ) AMG of 10-day-old Sox21a flies stained for 10xSTAT-GFP D (green) shows increased JAK/STAT activity in the tumour (indicated by a star). ( b ) AMG containing GFP-labelled Sox21a mutant clone stained for dpERK (red) at 16 days ACI. dpERK staining is observed around the Sox21a clone. ( c ) Tumour burden of flies with the indicated genotypes kept at 25 °C (mutant analysis) or 29 °C (overexpression analysis) for 21 days. Enh::Sox21a is a rescue construct with Sox21a under the control of its own enhancer sequence. ‘ EB >’ refers to the EB driver GBE TS , and ‘ EC> ’ refers to the enterocyte driver Myo1A TS . Numbers of flies scored for each genotype are indicated. ( d , e ) Expressing GFP ( d , control) or upd2-RNAi ( e ) in EBs of Sox21a flies placed for 21 days at 29 °C. Gut was stained with Armadillo (Arm; red, plasma membrane for progenitors) and Prospero (Pros, red, nuclear, for enteroendocrine cells). EBs are marked by GBE>GFP (green). ( f-g ) AMG of flies depleted for Notch ( N ) alone ( f ) or in combination with upd2 ( g ) for 4 days at 29 °C. The expression of upd2-IR in progenitors reduced tumour formation. ( h , i ) AMG of flies expressing GFP (control, h ) or upd2-RNAi ( i ) in the progenitor cells using the esg TS driver for 14 days at 29 °C shows that upd2 is required for basal stem cell maintenance. Progenitors are shown by esg>GFP in green ( f – i ) and by Arm immunostaining ( h , i ). P values in c (repeated three times) from χ 2 -test (* P <0.05; ** P <0.01; *** P <0.001). Each other individual image shown in a , b and ( d – i ) represents 20 flies tested in one experiment repeated three times. Full size image EB-derived Upd2 is essential for Sox21a tumour growth ISC proliferation can be induced upon expression of secreted ligands of the EGFR pathway (Spitz, Vein and Keren), the JAK-STAT pathway (unpaired 1, 2 and 3) and the Wingless pathway (Wg) [6] , [23] , [24] , [28] , [30] , [31] . To identify the factor stimulating stem cell division in Sox21a tumour, we applied a candidate gene approach by knocking down genes encoding these ligands in either EBs with GBE TS or in enterocytes with Myo1A TS . Depletion of the JAK/STAT ligand upd2 by RNAi in EBs but not in enterocytes strongly reduced tumour formation in Sox21a flies ( Fig. 4c–e ). Similarly, upd2; Sox21a -double mutant flies displayed a reduction in tumour burden ( Fig. 4c ). In contrast, inhibiting the other factors in EBs or enterocytes (Upd1, Keren and Wg) did not impair Sox21a tumour formation ( Supplementary Fig. 8a,b ). It should be noted that upd3 mutation and to a lesser extent depletion of Spitz in EBs had a modest effect on Sox21a tumours ( Fig. 4c ; Supplementary Fig. 8a ). This indicates that ISC proliferation is mostly induced by Upd2 released from Sox21a EBs composing the tumour. The stimulation of ISC proliferation by EB-derived Upd2 produces more differentiation-defective EBs, providing a feed-forward loop underlying the expansion of Sox21a tumours. We hypothesize that tumours are initiated in Sox21a flies upon stochastic clustering of EBs, leading to local increase of the mitogen Upd2. This mechanism would explain the random localization of tumours observed in the anterior midgut of Sox21a flies. In addition to Sox21a mutation, loss of Notch signalling in progenitors has been shown to induce tumours in the Drosophila midgut [14] , [15] , [32] . In contrast to the Sox21a EB tumours, Notch tumours are composed of ISCs that fail to differentiate into EBs. We have investigated the role of Upd2 in Notch tumour formation. Simultaneous depletion of upd2 and Notch by RNAi in the progenitors also suppressed Notch tumours ( Fig. 4f,g ), further emphasizing the role of Upd2 in tumour growth. Importantly, silencing upd2 in progenitor cells in an otherwise wild-type background led to a decrease in ISC numbers, pointing to a role of Upd2 in basal level stem cell maintenance ( Fig. 4h–i ). Mmp2 is required for Sox21a tumour progression We then investigated how a defect in the differentiation program transforms EBs into an aggressive tumour. For this, we compared gene expression of fluorescence-activated cell sorting (FACS)-sorted EBs of wild-type and Sox21a flies by RNA-seq [33] ( Fig. 5a ). Of 1,080 differentially expressed genes ( P <0.05, Robinson and Smyth Exact Test), 668 genes were reproducibly upregulated and 412 genes downregulated in Sox21a EBs compared with control ( Fig. 5b ). Gene ontology analysis of the RNA-seq data set revealed enrichment in genes involved in epithelia tube morphogenesis and redox homeostasis in Sox21a EBs ( Fig. 5c ). Many genes that were previously shown to be associated with tumorigenesis in other models were also identified in Sox21a tumour. For instance, the genes ImpL2 , an insulin/insulin-like growth factor antagonist recently reported to mediate tumour-induced organ wasting [34] , [35] , and p53 , which reprograms tumour metabolism [36] , were both upregulated in Sox21a EBs ( Fig. 5d ). Increased expression of breathless /fibroblast growth factor receptor (FGFR; btl ) in Sox21a EBs was confirmed using btl-Gal4 UAS-actGFP (referred to as btl>actGFP ; Supplementary Fig. 9a–f ). While btl>actGFP never labels intestinal cells in wild-type midgut ( Supplementary Fig. 9a ), expression of the btl>actGFP reporter was observed in the anterior but not posterior midgut of Sox21a flies, in regions where tumours form ( Supplementary Fig. 9b–f ). The observation that some but not all the Sox21a EBs express btl>actGFP highlights the cellular heterogeneity of Sox21a tumours ( Supplementary Fig. 9c ). 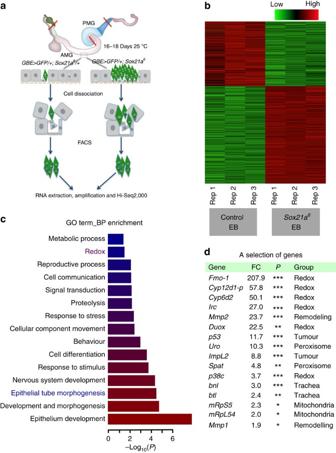Figure 5: EB-specific transcriptomics. (a), Transcriptional profiling ofSox21a/+(control) andSox21aEBs by RNA-seq was performed with messenger RNA isolated from FACS-sorted EBs based on the presence ofGBE>GFPfluorescent signal (see Method part for details). (b) Clustering of 1,080 differentially expressed genes (P<0.05, Robinson and Smyth exact test) betweenSox21a/+andSox21aEBs revealed that biological repeats (triplicates) cluster together. Columns correspond to replicate and rows to different genes. Relative expression level is indicated by the colour key shown at the top. (c) The 1,080 genes with differential expression were classified based on their gene ontology (GO) terms for biological process (BP). Enrichment of each GO term is shown with thePvalue. Red terms are the most significantly enriched ones. Redox and epithelial tube morphogenesis, described afterwards in the paper, are in red and blue, respectively. (d) A selection of genes upregulated inSox21aEBs. Fold change (FC), the range ofPvalues (*<0.05; **<0.01; ***<0.001) and the gene function groups are shown. Figure 5: EB-specific transcriptomics. ( a ), Transcriptional profiling of Sox21a/+ (control) and Sox21a EBs by RNA-seq was performed with messenger RNA isolated from FACS-sorted EBs based on the presence of GBE>GFP fluorescent signal (see Method part for details). ( b ) Clustering of 1,080 differentially expressed genes ( P <0.05, Robinson and Smyth exact test) between Sox21a/+ and Sox21a EBs revealed that biological repeats (triplicates) cluster together. Columns correspond to replicate and rows to different genes. Relative expression level is indicated by the colour key shown at the top. ( c ) The 1,080 genes with differential expression were classified based on their gene ontology (GO) terms for biological process (BP). Enrichment of each GO term is shown with the P value. Red terms are the most significantly enriched ones. Redox and epithelial tube morphogenesis, described afterwards in the paper, are in red and blue, respectively. ( d ) A selection of genes upregulated in Sox21a EBs. Fold change (FC), the range of P values (*<0.05; **<0.01; ***<0.001) and the gene function groups are shown. Full size image Interestingly, genes encoding two matrix metalloproteinases, matrix metalloproteinase 2 ( Mmp2 ) and to a lesser extent matrix metalloproteinase 1 ( Mmp1 ) were upregulated in Sox21a EBs ( Fig. 5d ). Use of an endogenous Mmp2-GFP fusion [37] confirmed an increased expression of Mmp2 specifically at the tumour site ( Fig. 6a,b ). Mmp1 and Mmp2 are downstream effectors of the JNK pathway that mediate tumour invasiveness in an imaginal disc tumour model [38] , [39] , [40] . Inactivating the JNK pathway by expressing a dominant-negative form of JNK ( basket, bsk ), depleting Mmp2 (but not Mmp1 ) or expressing the tissue inhibitor of metalloprotease ( timp ) in EBs of Sox21a flies reduced tumour burden and growth towards the lumen ( Fig. 6c–f ). Of note, Mmp2 but not Mmp1 was previously shown to be required for the invasive growth of larva air sac/trachea into tissues [41] . 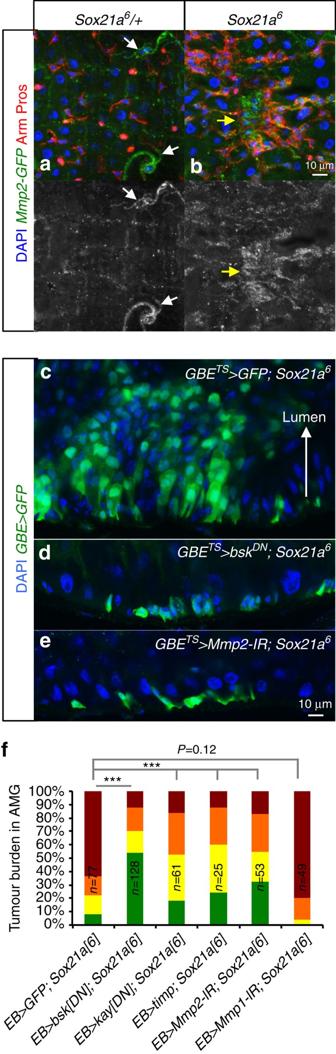Figure 6: Mmp2 is required for tumour progression. (a,b), Expression of Mmp2 detected with an endogenousMmp2-GFPfusion protein in the AMG of 10-day-oldSox21a/+(control,a) andSox21aflies (b). Arm (red, plasma membrane) and Pros (red, nuclear). Note that Mmp2 is only expressed in tracheal cells in the control (arrows in a), while it is expressed in the midgut progenitor cells (Arm positive) inSox21aflies (arrow inb). (c–e) Confocal sections ofSox21aintestines expressing GFP (control,c),bskDN(d) orMmp2-RNAi(e) in EB for 21 days at 29 °C. EBs are in green. (f), Tumour burden in AMG of flies with the indicated genotypes monitored at 21 days at 29 °C. Kayak (Kay) encodes the c-fos component of the JNK transcription factor AP-1.timpencodes a protein inhibitor of matrix metalloproteinase. Numbers of flies scored for each genotype (in biological triplicates) are indicated inf.Pvalues fromχ2-test (*<0.05; **<0.01; ***<0.001). Each other individual image shown ina–erepresents 20 flies tested in one experiment, which was repeated three times. Figure 6: Mmp2 is required for tumour progression. ( a , b ), Expression of Mmp2 detected with an endogenous Mmp2-GFP fusion protein in the AMG of 10-day-old Sox21a/+ (control, a ) and Sox21a flies ( b ). Arm (red, plasma membrane) and Pros (red, nuclear). Note that Mmp2 is only expressed in tracheal cells in the control (arrows in a), while it is expressed in the midgut progenitor cells (Arm positive) in Sox21a flies (arrow in b ). ( c – e ) Confocal sections of Sox21a intestines expressing GFP (control, c ), bsk DN ( d ) or Mmp2-RNAi ( e ) in EB for 21 days at 29 °C. EBs are in green. ( f ), Tumour burden in AMG of flies with the indicated genotypes monitored at 21 days at 29 °C. Kayak (Kay) encodes the c-fos component of the JNK transcription factor AP-1. timp encodes a protein inhibitor of matrix metalloproteinase. Numbers of flies scored for each genotype (in biological triplicates) are indicated in f . P values from χ 2 -test (*<0.05; **<0.01; ***<0.001). Each other individual image shown in a – e represents 20 flies tested in one experiment, which was repeated three times. Full size image Tumour progression requires JNK activation in enterocytes Tumour progression in Sox21a flies was associated with the elimination of neighbouring enterocytes, as shown by the progressive disappearance of 4,6-diamidino-2-phenylindole (DAPI)-stained polyploid cells ( Fig. 3g–j ; Supplementary Fig. 5a–d ). Tumour-induced elimination of normal cells has been observed in other cases and probably reflects a common feature of aberrantly proliferating cells [42] , [43] . It is reminiscent of cell competition in Drosophila , a type of short-range cell–cell interaction, where the fitter cells eliminate the unfit cells by activating JNK signalling [44] . Using a puckered enhancer trap ( puc-lacZ and puc-Gal4 ) as readout for JNK activity, we found that JNK signalling was induced in enterocytes surrounding Sox21a tumours from Sox21a flies or flies with EB-specific depletion of Sox21a by RNAi ( Fig. 7a,b ). Interestingly, JNK activation in enterocytes was coupled with the loss of the cell-polarity marker Discs large (Dlg) ( Fig. 7a ). In Notch ISC tumour [43] , flanking enterocytes are eliminated by delamination into the lumen. Similarly, confocal microscopy revealed the presence of delaminating enterocytes in the lumen of Sox21a flies at the vicinity of tumour ( Fig. 7c ). However, in Sox21a tumour, EBs were also found intercalated with enterocytes ( Fig. 7d ). Several observations indicate that JNK activation in enterocytes flanking Sox21a mutant tumours is essential for tumour progression. First, Sox21a flies lacking one copy of hemipterous ( hep ), a gene encoding the JNK kinase, have decreased tumour burden. In contrast, puc E69 /+ heterozygote flies with enhanced JNK activity display an increase of tumour burden of Sox21a flies ( Fig. 7e ). Second, inactivation of JNK signalling specifically in enterocytes by expressing a dominant-negative form of JNK greatly suppressed tumour formation and the presence of delaminating enterocytes ( Fig. 7e ). Moreover, the elimination of enterocytes nearby the tumours does not involve caspase-dependent apoptosis, as tumour progression was not affected by expressing the caspase inhibitor P35 ( Fig. 7e ). Collectively, our data show that Sox21a tumour progression involves the elimination of enterocytes by JNK activation independent of caspase activation. 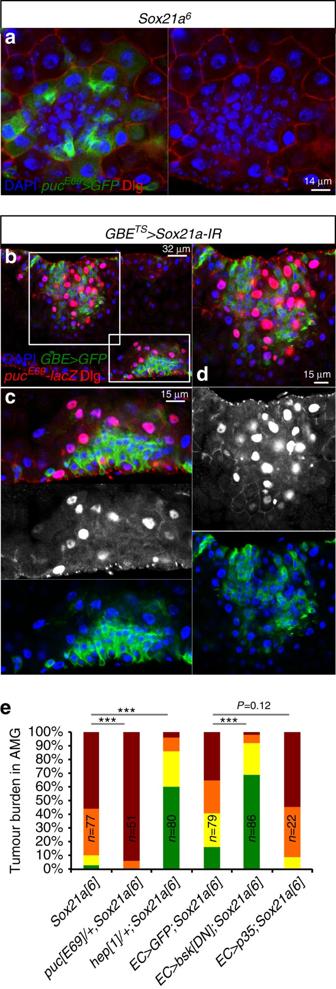Figure 7: Tumour-induced elimination of surrounding enterocytes requires JNK activation. (a) Two-week-oldSox21aintestine stained with the JNK activity reporterpucE69-Gal4 UAS-GFP(in green) and the basolateral cell-polarity marker Discs large (Dlg, in red). (b–d) Confocal section of intestine with EB-specific depletion ofSox21afor 2 weeks, stained with the JNK activity reporterpucE69-lacZ(red, nuclear) and Dlg (red, plasma membrane). EBs (GBE>GFP) are in green. (c,d) High-magnification view of two tumours defined inb. (e) Tumour burden in AMG of flies with the indicated genotypes monitored at 21 days. Flies were kept at 25 °C (for mutants) or 29 °C (for misexpression). Numbers of flies scored for each genotype (in biological triplicates) are indicated ine.Pvalues fromχ2-test (*<0.05; **<0.01; ***<0.001). Each other individual image shown ina–drepresents 20 flies tested in one experiment, which was repeated three times. Figure 7: Tumour-induced elimination of surrounding enterocytes requires JNK activation. ( a ) Two-week-old Sox21a intestine stained with the JNK activity reporter puc E69 -Gal4 UAS-GFP (in green) and the basolateral cell-polarity marker Discs large (Dlg, in red). ( b – d ) Confocal section of intestine with EB-specific depletion of Sox21a for 2 weeks, stained with the JNK activity reporter puc E69 -lacZ (red, nuclear) and Dlg (red, plasma membrane). EBs ( GBE>GFP ) are in green. ( c , d ) High-magnification view of two tumours defined in b . ( e ) Tumour burden in AMG of flies with the indicated genotypes monitored at 21 days. Flies were kept at 25 °C (for mutants) or 29 °C (for misexpression). Numbers of flies scored for each genotype (in biological triplicates) are indicated in e . P values from χ 2 -test (*<0.05; **<0.01; ***<0.001). Each other individual image shown in a – d represents 20 flies tested in one experiment, which was repeated three times. Full size image Increase of ROS activity at the vicinity of Sox21a tumour Reactive oxygen species (ROS) have been implicated in JNK activation and induction of cell death in Drosophila . For example, feeding flies with the ROS-generating compound Paraquat causes cellular damage and JNK activation in the midgut [45] , [46] . A recent study reported that ROS from apoptotic cells propagate to and activate JNK in the nearby cells [47] . This raises the possibility that tumour-derived ROS contribute to JNK activation in surrounding enterocytes, facilitating their elimination. We therefore investigated the role of ROS in tumorigenesis in Sox21a flies. Gene ontology analysis of the RNA-seq data set revealed enrichment in genes involved in redox homeostasis in Sox21a EBs ( Fig. 5c ). For instance, Sox21a EBs display increased expression of several Cytochrome P450 genes, the NADPH oxidase Dual oxidase ( Duox ) and its regulator, the MAPK p38c (refs 48 , 49 ), as well as several genes encoding mitochondria and peroxisome components ( Fig. 5d ). Mitochondria and peroxisomes are two main sources of intracellular ROS [50] . Using reporter constructs ( mitoGFP and peroxisome-GFP ), we observed an increase in mitochondrial and peroxisome signals at the tumour site, evocating a shift of metabolism ( Fig. 8a–e ; Supplementary Fig. 10a,b ). Increase of peroxisomes in Sox21a EBs is further supported by the expression of Catalase (Cat), a protein localized to peroxisome ( Fig. 8f,h ). Consistent with these observations, in vivo ROS detection using dihydroethidium (DHE) revealed a gradient of ROS peaking at the periphery of Sox21a tumours ( Fig. 8i ). Surprisingly, the level of ROS at the tumour site was lower, suggesting that EB tumour cells were less exposed to ROS compared with neighbouring enterocytes. Reporter genes and immunostaining analysis showed that many enzymes involved in ROS detoxification, including Catalase, Glutathione S -transferase D1 (GstD) and Superoxide dismutase 2 (SOD2) are enriched in progenitors of Sox21a flies ( Fig. 8g,h ; Supplementary Fig. 10c–e ). These observations suggest that these progenitor cells have an increased capacity to deal with ROS, and explain the lower level of ROS in Sox21a tumour. 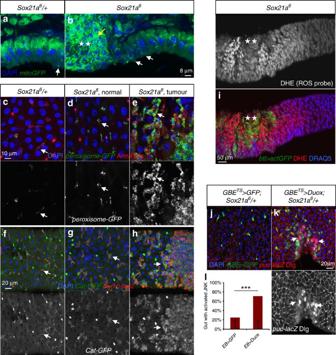Figure 8: Increase of ROS at the border ofSox21atumours. (a,b) Confocal sections of 2-week-oldSox21a/+(control,a) andSox21a(b) intestine expressing the mitochondrial-targeting GFP (mitoGFP, green) driven byAct5C-Gal4. WhilemitoGFP signals are found in progenitors of wild-type andSox21aflies (white arrows inaandb), a higher level of mitochondrial signal (yellow arrow inb) was observed at the site ofSox21atumour (indicated with two stars). (c–e,f–h) Two-week-oldSox21a/+(control,c,f) andSox21a(d,e,g,h) intestine either expressing a GFP fusion protein targeting the peroxisome (peroxisome-GFP, green) driven byAct5C-Gal4(c–e) or a Catalase (Cat)-GFP protein trap (f–h). Shown are regions from the AMG ofSox21aflies without (d,g) or with tumour (e,h). Signals corresponding to peroxisomes and Cat are both enriched in progenitor cells ofSox21aflies (Sox21a6, normal) compared with control flies (Sox21a6/+), and are further enhanced inSox21atumour sites (Sox21a6, tumour; indicated by arrows). Progenitors are marked by Arm (red, plasma membrane) inc–e. EBs are marked bySu(H)-lacZinf–h. (i) ROS distribution inSox21aintestine as revealed by dihydroethidium (DHE) staining of unfixed tissue. Cells are visualized by the live-cell DNA-dye DRAQ5 (blue) and tumour by the expression ofbtl>actGFP(green, indicated by two stars). (j–l) Representative images (j,k) and quantification (l) ofpuc-lacZexpression inSox21a/+flies either expressing GFP (control,j,l) orDuox(k,l) in EBs for 10 days at 29 °C. Examples of enterocyte with activated JNK signalling are indicated by arrows (k). Numbers of flies scored for each genotype (in biological triplicates) are indicated inl.Pvalues fromχ2-test (*P<0.05; **P<0.01; ***P<0.001). Each individual image shown ina–krepresents 12 flies tested in one experiment (in three biological replicates). Figure 8: Increase of ROS at the border of Sox21a tumours. ( a , b ) Confocal sections of 2-week-old Sox21a/+ (control, a ) and Sox21a ( b ) intestine expressing the mitochondrial-targeting GFP ( mitoGFP , green) driven by Act5C-Gal4 . While mitoGF P signals are found in progenitors of wild-type and Sox21a flies (white arrows in a and b ), a higher level of mitochondrial signal (yellow arrow in b ) was observed at the site of Sox21a tumour (indicated with two stars). ( c – e , f – h ) Two-week-old Sox21a/+ (control, c , f ) and Sox21a ( d , e , g , h ) intestine either expressing a GFP fusion protein targeting the peroxisome ( peroxisome-GFP , green) driven by Act5C-Gal4 ( c – e ) or a Catalase (Cat)-GFP protein trap ( f – h ). Shown are regions from the AMG of Sox21a flies without ( d , g ) or with tumour ( e , h ). Signals corresponding to peroxisomes and Cat are both enriched in progenitor cells of Sox21a flies ( Sox21a 6 , normal) compared with control flies ( Sox21a 6 /+), and are further enhanced in Sox21a tumour sites ( Sox21a 6 , tumour; indicated by arrows). Progenitors are marked by Arm (red, plasma membrane) in c – e . EBs are marked by Su(H)-lacZ in f – h . ( i ) ROS distribution in Sox21a intestine as revealed by dihydroethidium (DHE) staining of unfixed tissue. Cells are visualized by the live-cell DNA-dye DRAQ5 (blue) and tumour by the expression of btl>actGFP (green, indicated by two stars). ( j – l ) Representative images ( j , k ) and quantification ( l ) of puc-lacZ expression in Sox21a/+ flies either expressing GFP (control, j , l ) or Duox ( k , l ) in EBs for 10 days at 29 °C. Examples of enterocyte with activated JNK signalling are indicated by arrows ( k ). Numbers of flies scored for each genotype (in biological triplicates) are indicated in l . P values from χ 2 -test (* P <0.05; ** P <0.01; *** P <0.001). Each individual image shown in a – k represents 12 flies tested in one experiment (in three biological replicates). Full size image We then investigated the role of ROS in tumour formation by feeding Sox21a flies with an antioxidant, N -acetylcysteine amide (AD4). We observed that N -acetylcysteine amide-fed Sox21a flies have reduced tumour burden, although the difference with untreated control did not reach statistic significance ( Supplementary Fig. 8c ). Interestingly, overactivation of the ROS-producing enzyme Duox specifically in EBs of wild-type flies led to increased JNK activity in the flanking cells, and often resulted in local hyperplasia ( Fig. 8j–l ). In these experiments, foci of JNK activation were not observed around individual EBs but only around clustered EBs ( Fig. 8k ). Clustering of EBs expressing Duox might thus lead to a local increase of ROS above a threshold sufficient to trigger JNK activity. While the relevance of ROS in Sox21a tumour progression requires further investigation, our data raise the possibility that tumour-derived ROS non-cell autonomously contribute to JNK activation and elimination of flanking enterocytes. In this work, we report the functional characterization of a new regulator of ISC differentiation, introduce a novel tumour model and provide mechanistic insights on how tumour may arise from a simple defect in the differentiation program of stem cell progenies ( Fig. 9a,b ). 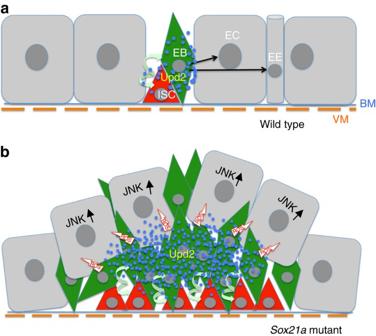Figure 9: Model ofSox21atumour initiation and progression. (a) Schematic representation of a wild-type intestinal epithelium. Intestinal stem cells (ISCs) are localized basally close to the basement membrane (BM) and visceral muscles (VMs). ISCs self-renew and differentiate to generate differentiating progenitors, the enteroblasts (EBs), which will then further differentiate into either enterocytes (ECs) or enteroendocrine (EE) cells. Progenitors express Upd2 (blue dots) stimulating basal level ISC turnover. (b) TheSox21amutation blocks the differentiation of EBs to ECs or EE cells, resulting in the accumulation of EBs. Clustered EBs create a centre with high Upd2 level that simulates ISCs division, generating more differentiation-defective EBs. EB tumour cells eliminate flanking ECs by delamination probably under the action of ROS and mechanical pressure. Elimination of flanking ECs, a process requiring JNK signalling activation, further provides space and mitogens allowing tumour progression. Figure 9: Model of Sox21a tumour initiation and progression. ( a ) Schematic representation of a wild-type intestinal epithelium. Intestinal stem cells (ISCs) are localized basally close to the basement membrane (BM) and visceral muscles (VMs). ISCs self-renew and differentiate to generate differentiating progenitors, the enteroblasts (EBs), which will then further differentiate into either enterocytes (ECs) or enteroendocrine (EE) cells. Progenitors express Upd2 (blue dots) stimulating basal level ISC turnover. ( b ) The Sox21a mutation blocks the differentiation of EBs to ECs or EE cells, resulting in the accumulation of EBs. Clustered EBs create a centre with high Upd2 level that simulates ISCs division, generating more differentiation-defective EBs. EB tumour cells eliminate flanking ECs by delamination probably under the action of ROS and mechanical pressure. Elimination of flanking ECs, a process requiring JNK signalling activation, further provides space and mitogens allowing tumour progression. Full size image Our data show that Sox21a, a previously uncharacterized transcription factor of the SOX family, plays a major role in the terminal differentiation of ISC progenies. Although the Drosophila genome encodes eight Sox genes, Sox21a is the only one enriched in the midgut. Sox21a is specifically expressed in progenitor cells along the entire midgut, and acts downstream of the JAK/STAT signalling to permit the transformation of EBs into enterocytes and enteroendocrine cells. Although Sox21a is required for both differentiated cell types, overexpression of Sox21a drives differentiation into enterocytes. It cannot be excluded that high level of Sox21a due to overexpression approach favours enterocyte rather than the enteroendocrine cell fate. Overexpression of Sox21a rescues the differentiation marker Pdm1 that is lost in JAK/STAT-deficient clones, demonstrating that Sox21a contributes significantly to EB differentiation downstream of this pathway. Consistent with this notion, our RNA-seq analysis demonstrates that Sox21a regulates a large set of genes including Pdm1 , which encodes a transcription factor involved in the terminal differentiation of enterocytes [20] . Our study also shows that Sox21a contributes to stem cell division notably in the posterior midgut. This is similar to the JAK/STAT pathway that impacts both stem cell division and differentiation [23] , [24] , [25] . The observation that Sox21a flies are viable indicates that the role of Sox21a is likely restricted to the adult intestinal homeostasis. Moving on, functional characterization of Sox21a target genes and identification of Sox21a-binding sites are now required to better understand the role of this transcription factor in ISC proliferation and progenitor differentiation. An unexpected observation of our work was that Sox21a flies developed tumours that increase in size and grow towards the intestinal lumen over time. Sox21a tumours are mainly composed of post-mitotic progenitors, the EBs that are blocked in their differentiation. Our study shows that the growth of Sox21a tumours relies on ISC division. The requirement for ISC proliferation to drive Sox21a tumours explains why tumours are not observed in the posterior midgut and are more frequent when flies are infected with bacteria, a condition that stimulates stem cell proliferation. Our results indicate that the release of a mitogen, Upd2, by accumulating EBs provides a feed-forward loop stimulating ISCs to divide and differentiate, leading to a further increase in the number of EBs. It is likely that Sox21a tumours are initiated at random sites where EB clustering leads to a local increase of Upd2. Like other cancer model, Sox21a tumours also express matrix metalloproteinase, which probably shapes the tumour local environment to promote tumour progression. Accumulating EBs display a shift in metabolism with an increased expression of ROS-producing factors, such as Duox and a higher number of mitochondria and peroxisomes. This metabolic shift is likely to underlie the increase of ROS at the vicinity of the tumour. We observed that the progenitors express at high-level ROS detoxification enzymes. Thus, the concomitant high-level synthesis of ROS and detoxifying enzymes by accumulating EBs restricts high ROS levels to the tumour borders. It is likely that ROS production promotes Sox21a tumour growth by eliminating flanking enterocytes in a JNK-dependent manner. Further experiments are required to determine whether JNK activation in flanking enterocytes is induced by ROS or by mechanical constraints from the tumours or by simultaneously both processes. Our tumour model introduces a new concept highlighting the active role of differentiating stem cell daughters in tumour formation. This model highlights the tumorigenic properties of transit differentiating cells and is in contrast to the current paradigm that emphasizes exclusively on the role of stem cells. In light of our findings, we speculate that the plasticity of these differentiating cells underlies their cancerous properties. Mechanistic studies of several intestinal tumour models have been reported previously in Drosophila [29] , [43] , [51] , [52] , [53] , [54] , [55] . The Sox21a tumour model is unique in its simplicity compared with other models that require complex genetic manipulations (for example, Ras V12 Scrib −/− (refs 56 , 57 ). Similar to Notch loss-of-function tumour model [43] , it reveals how a differentiation defect in the stem cell progenies can drive tumorigenesis. Both models are caused by a defect in the stem cell differentiation program, rely on stem cell division, and involve the elimination of flanking enterocytes by delamination through the JNK pathway. There are, however, major differences. First, Notch tumours are caused by a blockage of differentiation at the ISC stage [14] , [15] , [32] , while Sox21a is required later in the differentiation of EBs. This explains their distinct dynamics of tumour formation. Compared with the acute formation of Notch ISC tumour, the formation of Sox21a EB tumour is a slow and stochastic process. While Notch tumours can be observed only a few days after induction of Notch -deficient cells, >20 days is required to observe grade 3 tumours in Sox21a flies. Second, the growth of Notch tumour relies on the autocrine EGF ligand Spitz [43] and the JAK/STAT ligand Upd2 (our data), while the growth of Sox21a tumour requires the paracrine Upd2, and to a much lesser extent Spitz from EBs. Third, Sox21a tumours display a higher level of cellular heterogeneity, which has not been described for Notch tumours. Fourth, Sox21a tumours are not formed in mosaic intestine where Sox21a is mutated clonally, while Notch -deficient stem cells can grow into tumour in clones. Finally, our study uncovers a non-cell autonomous effect of ROS in tumour progression caused by metabolic changes in the tumour cells. The implication of ROS in cancer is an emerging theme of research. Thus, our model is likely to serve as a useful tool to study how ROS could play a signalling role to mediate short-range communication between tumour cells and their neighbours. Many human tumours are composed of cells with different degrees of differentiation, including differentiating progenitors derived from stem cells [11] . Our study highlights the cancerous properties of the differentiating stem cell progenies, which can stimulate stem cells proliferation and display a high cellular plasticity. Promoting the terminal differentiation of cancer cells has long been proposed and studied as a promising therapeutic strategy [58] . With increasing knowledge of genetic control of stem cell differentiation, it would be interesting to explore whether modulating progenitor cell differentiation can combat the progression of cancers. Tumour-burden quantification and statistical analysis Tumour burden of flies with different genotypes was quantified as follows. Flies were grown either at 25 °C (for mutant analysis) or at 18 °C (for overexpression analysis) until adulthood. Sorted genotypes were kept at 25 °C (for mutant analysis) or at 29 °C (for overexpression analysis) for 20–22 days. The midguts of flies were dissected and scored for tumour burden based on the criteria described below. Grade 0 midguts carried no tumour (Grade 0) and had progenitor cells that were evenly interspersed by large-nucleated enterocytes ( Fig. 3g,k ). Midguts with cluster of progenitor cells spanning 3–4 enterocytes were designated grade 1 ( Fig. 3h,l ). Large tumour mass and multilayering cells growing towards the lumen were features of grade 2 and 3 tumours. While enterocytes were still present in grade 1 and 2 tumours, grade 3 tumours were only composed of progenitors. Tumour border was defined as the place where the density of small-nucleated cells reduces to normal. The enterocytes surrounded by the grade 1 and 2 tumour cells were in the process of being eliminated through JNK activation, and we did not count them as part of the tumour. When a fly gut harboured several tumours, we assigned the final grade to the tumour with the highest grade. Overall, 20–30 flies were scored for each experiment and each experiment was repeated for at least three times. The results were pooled to generate graphs of tumour grade distribution in Excel. P values were calculated using χ 2 -test, and indicated with * P <0.05; ** P <0.01; or *** P <0.001. To test the effect of bacterial infection on tumour burden, Gram-negative bacteria Erwinia carotovora 15 ( Ecc15 ) was orally ingested by 7-day-old Sox21a flies at OD 600 =100. The flies were returned to normal food after 2 days on Ecc15 -containing medium, and scored for tumour burden after recovery for another 7 days. Other significance tests in the paper were done with Student’s t -test using the Prism 5 software. Drosophila strains Drivers : esg-Gal4, tub-Gal80 TS , UAS-GFP (referred to as esg TS ) [15] ; Myo1A-Gal4, tub-Gal80 TS , UAS-GFP (referred to as Myo1A TS ) [23] ; Su(H)GBE-Gal4, UAS-CD8::GFP; tub-Gal80 TS (referred to as GBE TS ) [17] ; Su(H)GBE-Gal4, UAS-nlsGFP, tub-Gal80 TS (referred to as GBE TS , this study); Dl-Gal4, UAS-GFP, tub-Gal80 TS (referred to as Dl TS ) [19] ; Act5C-Gal4 (BDSC25374); MARCM tester FRT2A: y,w,hsFlp; tub-Gal4, UAS-CD8::GFP; FRT2A, tub-Gal80 (gift from Yanrui Jiang) and y,w,hsFlp, tub-Gal4, UAS-nlsGFP;;FRT2A, tub-Gal80 (this study); MARCM tester FRT82B: y,w,hsFlp, tub-Gal4, UAS-nlsGFP;;FRT82B, tub-Gal80 (gift from Ernesto Sánchez-Herrero); GMR43E09-Gal4 (BDSC46247); puc E69 -Gal4 (ref. 59 ), miR-8-Gal4 NP5247 (DGRC104917) and btl-Gal4, UAS-actGFP (BDSC8807). Reporters : Su(H)-lacZ (ref. 60 ); puc-lacZ E69 (DGRC109029); Dl-lacZ (gift from Michael Boutros); gstD-lacZ (ref. 61 ); 10xstat-GFP D (ref. 62 ); Mmp2-GFP (BDSC60512); Dl-GFP (BDSC59819); Cat-GFP (BDSC51546); sqh-EYFP-Mito (BDSC7194). Mutants : upd2 Δ , upd3 Δ , and upd2-3 Δ (ref. 63 ); FRT82B, Stat 397 and hep 1 . UAS lines : UAS-hop tumL (gift from James Castelli-Gair Hombría); UAS-Stat-RNAi (BDSC35600); UAS-Sox21a-RNAi (HMJ21395 and HMJ21325); UAS-N-RNAi (VDRC100002); UAS-bsk DN (BDSC6409); UAS-kay DN (BDSC7214); UAS-timp, UAS-Mmp1-RNAi , and UAS-Mmp2-RNAi (ref. 38 ); UAS-P35 (BDSC5072); UAS-EGFR DN (BDSC5364); UAS-GFP.SKL (BDSC28881), UAS-mito-HA-GFP (BDSC8442); UAS-Sox21a (this study); UAS-spi-RNAi (VDRC103817); UAS-krn-RNAi (VDRC104299); UAS-wg-RNAi (VDRC13351 and 104579); UAS-upd1-RNAi (VDRC3282); UAS-upd2-RNAi (BDSC33949 and NIG5988R1-3) and UAS-upd3-RNAi (gift from Hervé Agaisse). The following lines were recombined to Sox21a 6 by mitotic recombination: FRT2A , Dl-lacZ , Dl-GFP , Cat-GFP , puc-lacZ , puc E69 -Gal4 , tub-Gal80 TS , UAS-timp and UAS-Mmp2-RNAi. Full genotypes of flies used in this study are listed in Supplementary Table 1 . In most of our experiments, we used Sox21a 6 /+ flies as control. We did not see any difference between Sox21a 6 /+ flies and wild-type flies, indicating that Sox21a 6 is a recessive mutation. Conditional expression of UAS-linked transgenes The TARGET system was used in combination with the indicated Gal4 drivers to conditionally express UAS-linked transgenes [64] . Flies were grown at 18 °C to limit Gal4 activity. After 3–5 days at 18 °C, adult flies with the appropriate genotypes were shifted to 29 °C, a temperature inactivating the temperature-sensitive Gal80’s ability to suppress Gal4. MARCM clone induction The Sox21a 6 allele was recombined to FRT2A site for MARCM analysis [22] . For clone induction, 3–5-day-old flies with the appropriate genotypes were heat-shocked for 30 min at 37.5 °C in a water bath. The flies were immediately transferred into a new tube and kept at 25 °C until dissection. Rescue experiments were performed by combining the UAS-Sox21a transgene with the FRT2A , Sox21a 6 or FRT82B , Stat 397 chromosome. Note that UAS-Sox21a was only expressed in the clones indicated by the presence of GFP. Generation of Sox21a mutant and transgenes Sox21a mutant flies were generated with the method described before [21] with the guide RNA sequence: 5′- GCTTTCATGGTCTGGTCGCG -3′. The alleles originally named Sox21a SK6 and Sox21a SK8 were referred to as Sox21a 6 and Sox21a 8 in the paper. To generate the enh:: Sox21a construct, the following primers (5′- caccATGACGAGCATCTCGGCCCTG -3′ and 5′- TCAAATGATGTTTGGCGGACT -3′) were used to amplify the 2.8-kb Sox21a-RA -coding regions together with the intronic Sox21a enhancer from the genomic DNA of a wild-type fly. The PCR product was first cloned into pENTR-D-TOPO (Life Technologies) vector, and then swapped into either pTW destination vector to make UAS-Sox21aEnh::Sox21a or pTRW destination vector to make UAS-RFP-Sox21aEnh::Sox21a . Transgenic flies were established by standard P element-mediated germline transformation. At least three independent lines of each construct were tested for expression level. Note that without the presence of a Gal4 activator, the UAS-RFP-Sox21aEnh::Sox21a transgene drives the RFP reporter under the control of Sox21a cis -regulatory sequence. Despite the presence of RFP, this construct can rescue the Sox21a mutation ( Fig. 4c ). Histology and immunostaining Flies were transferred overnight into a classical fly food vial containing a filter paper soaked with a solution consisting of 5% sucrose to clear the digestive tract. Then, guts of adult females were dissected in PBS, and fixed for at least 1 h at room temperature in 4% paraformaldehyde in PBS. They were subsequently rinsed in PBS+0.1% Triton X-100 (PBT), permeabilized and blocked in 2% bovine serum albumin PBT for 1 h, and incubated with primary antibodies in 2% bovine serum albumin PBT for overnight at 4 °C. After 1-h washing, secondary antibodies and DAPI were applied at room temperature for 2 h. Phalloidin was added to the secondary antibody incubation step in some experiments. Histology and staining on cross-sectioned guts were done as described previously [65] . For ROS measurement with DHE, guts were dissected and directly incubated in 30 μM DHE (Life Technologies) and DRAQ5 (BioStatus, 1:200) for 10 min at room temperature, washed twice and mounted for confocal microscopy immediately. GFP expressed under the control of btl>actGFP was used to identify the location of tumour, and live-cell dye DRAQ5 was used to visualize all the cells. Primary antibodies used are as follows: mouse anti-Pros (DSHB, 1:100), mouse anti-Arm (DSHB, 1:100), mouse anti-Dlg (DSHB, 1:100), rabbit anti-Pdm1 (1:500, gift from Xiaohang Yang), rabbit anti-pH3 (Millipore, 1:1,000), chicken anti-GFP (Abcam, 1:1,000) and rabbit anti-βGal (Cappel, 1:1,000). Alexa488-, Alexa555- or Alexa647-conjugated secondary antibodies (Life Technologies) were used. Nuclei were counterstained by DAPI (Sigma), and Alexa555 Phalloidin (Life Technologies) was used to stain F-actin. All the images were taken on a Zeiss LSM 700 confocal microscope, except the whole gut on the Olympus slide scanner. Images were processed using Image J and Adobe Photoshop software. Shown in figures are the maximal intensity projections of all the z -stacks taken with the confocal, in the same orientation (anterior to the left, and posterior to the right). FACS and RNA-seq Crosses were set-up at 25 °C to obtain Sox21a/+ (used as control) or homozygous Sox21a flies carrying the GBE>CD8::GFP transgenes. Eclosed flies were maintained at 25 °C for 16–18 days. Around 150 flies for each biological replicate were dissected in ice-cold 1 × PBS made with diethylpyrocarbonate (DEPC)-treated water under a dry-ice chilled dissecting microscope, within a 1-h time frame. Proventriculus, hindgut and midgut/hindgut junction were removed to collect only midgut GBE>CD8::GFP -positive cells. Trimmed midguts were split in the copper cell region of the middle midgut to obtain both the anterior midgut and the posterior midgut. Three biological replicates were performed. Cell dissociation, FACS sorting, total RNA isolation and messenger RNA amplification were performed according to the method described before [33] . Elastase solution with a final concentration of 1 mg ml −1 was used for cell dissociation. Cells positive for GFP and negative for propidium iodide were directly sorted into a tube containing RNA extraction buffer on a BD FACSAria II cell sorter. RNA was isolated using the Arcturus PicoPure RNA Isolation Kit (Life Technologies). Messenger RNA was amplified using a two-step linear amplification protocol with the Arcturus RiboAmp HS Plus RNA Amplification Kit (Life Technologies), with 2 ng total RNA as input. We usually obtained >100-μg amplified antisense RNA. Amplified antisense RNA integrity was determined with an Agilent 2100 Bioanalyzer before complementary DNA library preparation with the TruSeq RNA Sample Prep Kit-v2 (Illumina). RNA-seq was performed on a Hi ‐ Seq2000 (Illumina) with 100 nt paired ‐ end sequencing. RNA-seq data have been deposited in GEO under the accession number GSE71093. RNA-seq data analysis Pair-end reads were mapped to the Drosophila melanogaster genome (release version 6.02) using Bowtie2 (ref. 66 ) with forward and reverse composition. Each sequencing experiment generated in total >40 million raw reads, and >80% was successfully mapped for each experiment. Gene expression was quantified by the number of paired reads that fall into the exons. Normalization was carried out using the size factor formula [67] . Differentially expressed genes were identified using the method as described [68] . Over-represented gene ontology (GO) terms were computed by PANTHER [69] . GO terms were further filtered if the observed number of genes was <5% of the total input number of genes, and 25% of GO terms were discarded according to the ranking of fold enrichment. qRT–PCR primers Sox21a_F : 5′- GGACAGAAGCGTCCATTCAT -3′; Sox21a_R : 5′- TGACTTGTTGAGCGTCTTGG -3′ RpL32_F : 5′- TCTGCATGAGCAGGACCTC -3′; RpL32_R : 5′- ATCGGTTACGGATCGAACAA -3′. How to cite this article: Zhai, Z. et al . Accumulation of differentiating intestinal stem cell progenies drives tumorigenesis. Nat. Commun. 6:10219 doi: 10.1038/ncomms10219 (2015).